RETRACTED ARTICLE: A switch in the poly(dC)/RmlB complex regulates bacterial persister formation Bacterial persisters are phenotypic variants that tolerate exposure to lethal antibiotics. These dormant cells are responsible for chronic and recurrent infections. Multiple mechanisms have been linked to persister formation. Here, we report that a complex, consisting of an extracellular poly(dC) and its membrane-associated binding protein RmlB, appears to be associated with persistence of the opportunistic pathogen Pseudomonas aeruginosa . Environmental stimuli triggers a switch in the complex physiological state (from poly(dC)/RmlB to P-poly(dC)/RmlB or RmlB). In response to the switch, bacteria decrease proton motive force and intracellular ATP levels, forming dormant cells. This alteration in complex status is linked to a (p)ppGpp-controlled signaling pathway that includes inorganic polyphosphate, Lon protease, exonuclease VII (XseA/XseB), and the type III secretion system. The persistence might be also an adaptive response to the lethal action of the dTDP- l -rhamnose pathway shutdown, which occurs due to switching of poly(dC)/RmlB. Bacterial persisters are dormant cells that form stochastically within isogenic bacterial populations. These transient and non-hereditary phenotypic cells are highly tolerant to lethal doses of antibiotics and have been suggested as causative agents of chronic and recurrent infections [1] . Unlike normal vegetative cells (majority of cells in a population), persisters (minority of cells in a population) remain viable in the presence of antibiotics. Furthermore, following antibiotic withdrawal the dormant cells resume growth and infection [1] , [2] , [3] , [4] . The transient nature of persistence makes this phenomenon inherently difficult to study; therefore, many of the molecular mechanisms that underlie persistence remain to be elucidated. Most of what we know about mechanisms pertaining to persister formation comes from studies associated with human pathogens [4] , [5] , [6] . Prokaryotic toxin/antitoxin (TA) modules have been reported as important effectors of persistence since TA module expression is known to cause the shutdown of important cellular processes, thereby inducing dormancy [7] , [8] , [9] , [10] , [11] , [12] , [13] , [14] , [15] , [16] , [17] . The stringent response alarmone (p)ppGpp and the ubiquitous Lon protease can drive persister formation under unstressed conditions [18] , [19] , [20] . Environmental stimuli, including DNA-damaging agents, oxidative and acid stress, heat shock, respiration inhibition, chemical signaling, carbon-source transitions, and ATP depletion also have an apparent role in the induction of persistence [4] , [6] , [21] , [22] , [23] , [24] , [25] , [26] , [27] . Additionally, several global regulators are reported to be associated with persistence [28] . Pseudomonas aeruginosa is an important opportunistic pathogen that causes severe infections in immunocompromised patients [29] . Apart from its intrinsic tolerance against antibiotics, the presence of persisters makes it difficult to treat infections from this pathogen [30] . The mechanisms that underlie P. aeruginosa persistence are heretofore not well understood. Two ubiquitous type II TA modules, namely RelBE and HigBA, are present in several P. aeruginosa clinical isolates [31] , [32] , [33] . The latter protein has been shown to contribute to persistence, but deletion of higB does not result in persistence phenotypic variants, suggesting the existence of other unknown switching mechanisms [32] , [33] . Furthermore, the quorum-sensing signaling molecules pyocyanin and acyl-homoserine lactone (acyl-HSL) are known to have an important role in the regulation of P. aeruginosa persister formation [34] . However, deletion of the pyocyanin biosynthetic pathway has no effect on persistence, further raising the possibility that additional signaling systems control the bacterial persistence phenotype [4] . In this study, we report a persistence-associated complex that directly controls persister formation in response to environmental stimuli in P. aeruginosa PAO1. The complex consists of an extracellular 5′-dephospho-polydeoxycytidylic acid (poly(dC)) and its membrane-associated binding protein RmlB. After removal of the DNA component, or switching of the complex to 5′-phosphorylated poly(dC)/RmlB (P-poly(dC)/RmlB) by in-situ DNA phosphorylation or tailoring (from the 5′ terminus), we observe significant decreases in proton motive force (PMF) across the membrane and in intracellular ATP levels with a concomitant increase in persistence. Spontaneous bacterial complex switching depends on a (p)ppGpp-controlled signaling pathway that contains inorganic polyphosphate (PolyP), Lon protease, exonuclease VII (XseA/XseB), and the type III secretion system (T3SS). Furthermore, the complex switching shuts down the dTDP- l -rhamnose pathway, thereby leading to lethality in cells. Thus, P-poly(dC)/RmlB- or RmlB-triggered persistence might also be deemed as an adaptive response to the detrimental effect. Bacterial persistence correlates with extracellular poly(dC) Previous studies have demonstrated that environmental insults can induce persister formation [4] , [6] , [19] , [20] , [21] , [22] , [23] , [24] , [25] . Here, we found that a routine procedure for washing cells increased persister levels 10 2 - to 10 3 -fold in exponential (i.e., 6 h) and stationary (i.e., 18 h) (hereafter called ( e ) and ( s )) wild-type (WT) P. aeruginosa PAO1, but not in WT Escherichia coli K-12 (Fig. 1a, b ; Supplementary Figs. 1 , 2 ). The procedure consisted of removal of medium by washing three times in sterile water (3 min centrifugation at 12,000 × g ) and resuspension of cells in fresh medium (with the same pH as that of spent medium) prior to antibiotic challenge (also see Methods). The centrifugation could not increase bacterial survival (Supplementary Fig. 3a, b ). In the meantime, the washing step did not result in a delay (an extended lag time) in cell regrowth or a positive response in antibiotic stress associated protein, both of which might account for the observed tolerance [35] (Supplementary Fig. 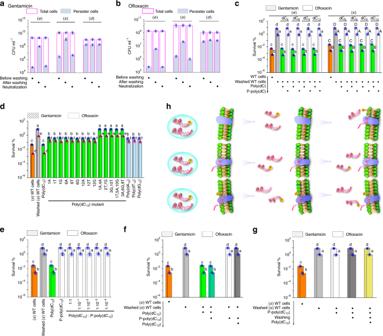Fig. 1 Extracellular poly(dC) modulates PAO1 persistence.a,bThe number of total and persister cells before and after washing (e), (s), or (d) WT cells as well as after resuspending corresponding washed cells in their native supernatants (neutralization).cPersistence in washed (e) WT cells or washed (s) WT cells plus short poly(dC) or P-poly(dC). Poly(dC) instead of P-poly(dC) reduced persistence in washed (e) WT cells and washed (s) WT cells.dPersistence in washed (s) WT cells plus each poly(dC12) mutant, poly(dA12), poly(dT12), or poly(dG12). These ssDNA led to a nearly 10-fold reduction in persistence of washed (s) WT cells. As a control, poly(dC12) caused a more than 100-fold reduction in persistence of washed (s) WT cells.ePersistence in washed (s) WT cells plus poly(dC12) and P-poly(dC12) with different molar ratios. P-poly(dC12) abolished the regulatory activity of poly(dC12) in persistence of washed (s) WT cells.fPersistence in washed (s) WT cells plus poly(dC12) for 10 min and then P-poly(dC12) for 10 min or plus P-poly(dC12) for 10 min and then poly(dC12) for 10 min. P-poly(dC12) did not regulate persistence in poly(dC12)-pretreated washed (s) WT cells and vice versa.gPersistence in washed (s) WT cells plus P-poly(dC12) for 10 min, washing again, and then plus poly(dC12) for 10 min. These treatments did not reduce persistence in washed (s) WT cells.hProposed model for functional antagonism between poly(dC) and P-poly(dC). All experiments were performed in biological triplicates. Error bars represent standard deviations. Dot plots overlaid on bar graphs represent individual data points. Black spot, treatment step or object; arrow, treatment order 3c ; Supplementary Table 1 ). Interestingly, the increase in persistence was neutralized by resuspension of the washed cells in their native supernatants (Fig. 1a, b ; Supplementary Fig. 1b, c ). The same persistence regulation phenomenon was also observed in a Δ(higBA relBE) mutant and a Δ(lasI rhlI) mutant (without acyl-HSL signals), suggesting the existence of an independent extracellular effector that modulates persister formation (Supplementary Figs. 4 , 5 ). Next, we assessed the possibility that chemical compounds, protein, RNA and DNA could act as potential effectors in ( e ) and ( s ) WT supernatants. To our surprise, DNA was the only stimulatory agent in both supernatants. Indeed, digestion of extracellular total DNA with DNase I abolished the regulation of persistence to washed cells by the supernatants (Supplementary Fig. 3d ). Digestion of extracellular single-stranded DNA (ssDNA) instead of double-stranded DNA (dsDNA) led to the same results (Supplementary Fig. 3e ). Conversely, ( e ) and ( s ) supplementation with extracellular ssDNA extracts recovered the regulatory activities associated with the DNA-free supernatants (Supplementary Fig. 3f ). These results suggest a crucial role for ( e ) and ( s ) extracellular ssDNA in washing-induced persister formation. Fig. 1 Extracellular poly(dC) modulates PAO1 persistence. a , b The number of total and persister cells before and after washing ( e ), ( s ), or ( d ) WT cells as well as after resuspending corresponding washed cells in their native supernatants (neutralization). c Persistence in washed ( e ) WT cells or washed ( s ) WT cells plus short poly(dC) or P-poly(dC). Poly(dC) instead of P-poly(dC) reduced persistence in washed ( e ) WT cells and washed ( s ) WT cells. d Persistence in washed ( s ) WT cells plus each poly(dC 12 ) mutant, poly(dA 12 ), poly(dT 12 ), or poly(dG 12 ). These ssDNA led to a nearly 10-fold reduction in persistence of washed ( s ) WT cells. As a control, poly(dC 12 ) caused a more than 100-fold reduction in persistence of washed ( s ) WT cells. e Persistence in washed ( s ) WT cells plus poly(dC 12 ) and P-poly(dC 12 ) with different molar ratios. P-poly(dC 12 ) abolished the regulatory activity of poly(dC 12 ) in persistence of washed ( s ) WT cells. f Persistence in washed ( s ) WT cells plus poly(dC 12 ) for 10 min and then P-poly(dC 12 ) for 10 min or plus P-poly(dC 12 ) for 10 min and then poly(dC 12 ) for 10 min. P-poly(dC 12 ) did not regulate persistence in poly(dC 12 )-pretreated washed ( s ) WT cells and vice versa. g Persistence in washed ( s ) WT cells plus P-poly(dC 12 ) for 10 min, washing again, and then plus poly(dC 12 ) for 10 min. These treatments did not reduce persistence in washed ( s ) WT cells. h Proposed model for functional antagonism between poly(dC) and P-poly(dC). All experiments were performed in biological triplicates. Error bars represent standard deviations. Dot plots overlaid on bar graphs represent individual data points. Black spot, treatment step or object; arrow, treatment order Full size image In order to further characterize the role of ssDNA molecules in the regulation of persistence, numerous ( e ) and ( s ) extracellular ssDNA molecules were sequenced and resynthesized as primers (Supplementary Data 1 ). We then tested the persistence regulatory activities of the primers and observed that only four short poly(dC) molecules, poly(dC 6 ), poly(dC 8 ), poly(dC 9 ), and poly(dC 12 ), exhibited similar regulatory activities as the afore-mentioned native supernatants. The synthetic primers caused a marked reduction (10 2 - to 10 3 -fold) in persistence of washed ( e ) WT cells and washed ( s ) WT cells, respectively (Fig. 1c ). A dose-dependent persistence reduction was present at the concentrations of primers from 10 −3 to 10 −6 μM (Supplementary Fig. 6 ). Long poly(dC) molecules were also observed in extracellular supernatants; however, we failed to elucidate their exact length due to strong signal attenuation during sequencing. Consequently, we randomly synthesized several long poly(dC) molecules from 20 to 40 bases in length. These long poly(dC) molecules exhibited the same regulatory activity and the dose-dependent persistence reduction as the shorter molecules, indicating that poly(dC) is potentially a length-independent effector (Supplementary Figs. 3g , 6 ). Interestingly, the synthesized poly(dC) molecules lack 5′-phosphate groups while native DNA usually contains these moieties. Thus, we measured the regulatory activity of P-poly(dC) during washing-induced persistence. Unexpectedly, P-poly(dC) did not reduce the persistence in washed ( e ) WT cells and washed ( s ) WT cells (Fig. 1c ). Moreover, 5′-phosphorylated ( e ) or ( s ) WT extracellular ssDNA extracts also failed to recover the regulatory activity of each DNA-free supernatant, indicating that potential effectors do not have 5′-phosphate groups (Supplementary Fig. 3f ). In addition, washing of poly(dC)-pretreated washed ( e ) WT cells and poly(dC)-pretreated washed ( s ) WT cells caused a 10 2 - to 10 3 -fold increase in persistence, suggesting that poly(dC) has the same effect on washed WT cells as the potential effector (Supplementary Fig. 3h ). Given all of these results, we identified poly(dC) as the target effector. We also found that the regulatory activity of poly(dC) is highly influenced by its base composition since random single base substitutions caused at least a 10-fold reduction in the regulatory activity of poly(dC 12 ) during persistence and random multi bases ( n ≥ 2) substitutions abolished its regulatory activity completely (Fig. 1d ). Interestingly, when all bases were substituted by dA, dG, or dT (these three molecules were not detected in extracellular ssDNA molecules), the regulatory activity was partially recovered with at least a 10-fold reduction compared to that of poly(dC 12 ) (Fig. 1d ). Functional antagonism between poly(dC) and P-poly(dC) In accordance with the conclusion that poly(dC) is a length-independent effector, modification of the length of poly(dC 12 ) with exonuclease I (partial digestion) did not affect its regulatory activity in relation to persistence (Supplementary Fig. 7a, b ). However, modification of the length of poly(dC 12 ) with DNase I (also partial digestion) resulted in the loss of regulatory activity (Supplementary Fig. 7a, b ). Given that the latter digestion resulted in P-poly(dC) whereas the former did not, we speculated that this unexpected result is caused by the phosphorylation of poly(dC). This hypothesis was supported by the observation that poly(dC 12 ) did not reduce persistence in washed ( s ) WT cells following addition of the cells to any of the synthesized P-poly(dC) molecules including P-poly(dC 6 ), P-poly(dC 12 ), and P-poly(dC 30 ); this observation was made even when the molar ratio was 1:10 −4 (poly(dC 12 )/P-poly(dC)) (Fig. 1e ; Supplementary Fig. 7c, d ). These results indicate that P-poly(dC) is a functional antagonist against native poly(dC). Remarkably, we did not observe this antagonism following addition of P-poly(dC 12 ) to ( s ) WT cells (which contained poly(dC)) (Supplementary Fig. 7e ). Thus, it would appear that P-poly(dC) cannot antagonize poly(dC) when poly(dC) is already present. To investigate this hypothesis, we measured the level of persistence in washed ( s ) WT cells that were pretreated with poly(dC 12 ) for 10 min following exposure to P-poly(dC 12 ). As expected, P-poly(dC 12 ) did not regulate persistence in the poly(dC 12 )-pretreated washed ( s ) WT cells (Fig. 1f ). Since P-poly(dC) antagonizes native poly(dC), P-poly(dC) should also antagonize the post-treatment poly(dC). This deduction was supported by the observation that poly(dC 12 ) failed to regulate persistence in washed ( s ) WT cells that had been pretreated with P-poly(dC 12 ) for 10 min (Fig. 1f ). Interestingly, after washing of the P-poly(dC 12 )-pretreated washed ( s ) WT cells, poly(dC 12 ) still did not reduce the persistence, indicating that washing cannot thoroughly eradicate P-poly(dC) from the cells (Fig. 1g ). Based on these observations, we proposed a model to help explain the antagonism (Fig. 1h ). P-poly(dC) might share a common binding site with poly(dC). When this site is empty, it would facilitate preferential P-poly(dC) binding, leading to antagonism against poly(dC). Poly(dC) could not replace the site-bound P-poly(dC), and vice versa. During bacterial growth, an increase in persistence and the associated resistance to poly(dC 12 ) post-treatment was observed in both death phase (i.e., 39 h) (hereafter called ( d )) WT cells and the corresponding washed cells (Supplementary Fig. 7f ). The results were consistent with the previous results from the P-poly(dC 12 )-pretreated washed ( s ) WT cells, raising the possibility that P-poly(dC) appears in the death phase. In relation to the afore-mentioned hypothesis, the presence of 5′-phosphate groups was confirmed by the observation that alkaline phosphatase-mediated dephosphorylation counteracted the enhancement of persistence in ( d ) WT cells and associated washed cells (Supplementary Fig. 7g, h ). The DNA sequence was subsequently identified in the alkaline phosphatase-treated washed ( d ) WT cells. After washing of these cells, we only detected short poly(dC) molecules such as poly(dC 4 ) and poly(dC 5 ) following elution. The combined results demonstrate that switching from poly(dC) to P-poly(dC) is a bacterial strategy in the modulation of persistence. According to the afore-mentioned model, P-poly(dC) does not directly replace site-bound poly(dC). Thus, our observations suggest the existence of an in-situ switching (in-situ processing bound poly(dC) to bound P-poly(dC)) mechanism for DNA. Membrane-associated protein RmlB is the common binding site A common binding site for the different DNA molecules was proposed above. As part of this study we also performed a two-part experiment involving Cy5-labeled P-poly(dC 12 ) (P-poly(dC 12 )*) and Cy5-labeled poly(dC 12 ) (poly(dC 12 )*) to identify the afore-mentioned site. The Cy5 fluorescent label was attached to the 3′ terminus and thereby did not affect the activity of either DNA molecule (Supplementary Fig. 8a ). In the first part, we added P-poly(dC 12 )* to washed ( s ) WT cells. A follow-up wash step removed the free-labeled DNA while leaving the intact bound-labeled DNA. In the second part, we added poly(dC 12 )* to washed ( s ) WT cells. An extra in-situ phosphorylation was introduced to prevent the loosely bound labeled DNA being extricated from the site in the following wash step. Subsequently, the bound-labeled DNA from each part was cross-linked to its associated binding site by formaldehyde. The fluorescent signals representing the binding site were separated from both membrane protein extracts by 2D-PAGE and finally identified as RmlB (locus tag, PA5161) by LC/MS (Supplementary Fig. 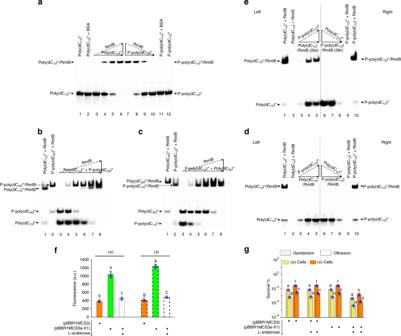Fig. 2 RmlB controls persistence in PAO1.aFormation of DNA/protein complex by RmlB binding poly(dC12)* or P-poly(dC12)*. In lanes 3–6, a constant concentration of poly(dC12)* and an increasing concentration of His-tagged RmlB were mixed together. In lanes 7–10, a constant concentration of P-poly(dC12)* and a decreasing concentration of His-tagged RmlB were mixed together.bOrder of RmlB binding poly(dC12)* and P-poly(dC30)*. In lanes 3–8, a constant concentration of poly(dC12)*/P-poly(dC30)* mixture and an increasing concentration of His-tagged RmlB were mixed together.cOrder of RmlB binding P-poly(dC12)* and poly(dC30)*. In lanes 3–8, a constant concentration of P-poly(dC12)*/poly(dC30)* mixture and an increasing concentration of His-tagged RmlB were mixed together.d,eSubstitutability of ssDNA in poly(dC12)/RmlB and P-poly(dC12)/RmlB. In lanes 3–5, a constant concentration of poly(dC12)/RmlB and an increasing concentration of P-poly(dC12)* were mixed together with (e) or without (d) vortex. In lanes 6–8, a constant concentration of P-poly(dC12)/RmlB and a decreasing concentration of poly(dC12)* were mixed with (e) or without (d) vortex.fRed fluorescence of cells harboring pBBR1MCS3a-X1 with or withoutl-arabinose induction. The RmlB fused with mCherry was expressed from a native promoter ofrmlBin pBBR1MCS3a-X1. It caused a 2.9-fold increase in fluorescence as compared to cells harboring pBBR1MCS3. Red fluorescence was decreased 2.47-fold upon expression ofrmlBasRNAfrom pBBR1MCS3a-X1 with 0.2%l-arabinose induction. The basal level of fluorescence with the empty vector (pBBR1MCS3) should come from the metabolites of bacteria. a.u. arbitrary units.gPersistence in cells harboring pBBR1MCS3a-X1 with or withoutl-arabinose induction. ExpressingrmlBasRNAwith 0.2%l-arabinose induction caused a nearly 24-fold decrease in persistence of the (e) or (s) cells. All experiments were performed in biological triplicates. Error bars represent standard deviations. Dot plots overlaid on bar graphs represent individual data points. Black spot, treatment step or object; arrow, treatment order 8b ; Supplementary Table 2 ). This result raises the possibility that the membrane-associated protein RmlB represents the common binding site for both DNA molecules. Next, we expressed and purified His-tagged RmlB and analyzed its ssDNA binding activity using an electrophoretic mobility shift assay (EMSA) (Fig. 2 ; Supplementary Fig. 8c ). ssDNA with a Cy5 label (*) attached to the 3′ terminus was used to visualize the binding reactions. His-tagged RmlB impeded the migratory capacity of the DNA/protein complex containing either poly(dC 12 )* or P-poly(dC 12 )* but failed to impede that of other ssDNA* without persistence regulatory activity (Fig. 2a ; Supplementary Fig. 8d, e ). Following incubation with a mixture of poly(dC 12 )*/P-poly(dC 30 )* or P-poly(dC 12 )*/poly(dC 30 )*, His-tagged RmlB preferentially complexed with P-poly(dC)* and only complexed with poly(dC)* after exhaustion of all P-poly(dC)* (Fig. 2b, c ). Furthermore, His-tagged RmlB did not permit the replacement of bound poly(dC 12 ) with P-poly(dC 12 )*. Therefore, the labeled slower migrating complex did not re-form unless the bound poly(dC 12 ) was stripped off by a rigorous stirring procedure (Fig. 2d (left), e(left)). Meanwhile, this protein did not allow poly(dC 12 )* to replace bound P-poly(dC 12 ) either, even when a vortex meter was used to attempt to disrupt the complex (Fig. 2d (right), e(right)). These observations were consistent with the afore-mentioned model. Fig. 2 RmlB controls persistence in PAO1. a Formation of DNA/protein complex by RmlB binding poly(dC 12 )* or P-poly(dC 12 )*. In lanes 3–6, a constant concentration of poly(dC 12 )* and an increasing concentration of His-tagged RmlB were mixed together. In lanes 7–10, a constant concentration of P-poly(dC 12 )* and a decreasing concentration of His-tagged RmlB were mixed together. b Order of RmlB binding poly(dC 12 )* and P-poly(dC 30 )*. In lanes 3–8, a constant concentration of poly(dC 12 )*/P-poly(dC 30 )* mixture and an increasing concentration of His-tagged RmlB were mixed together. c Order of RmlB binding P-poly(dC 12 )* and poly(dC 30 )*. In lanes 3–8, a constant concentration of P-poly(dC 12 )*/poly(dC 30 )* mixture and an increasing concentration of His-tagged RmlB were mixed together. d , e Substitutability of ssDNA in poly(dC 12 )/RmlB and P-poly(dC 12 )/RmlB. In lanes 3–5, a constant concentration of poly(dC 12 )/RmlB and an increasing concentration of P-poly(dC 12 )* were mixed together with ( e ) or without ( d ) vortex. In lanes 6–8, a constant concentration of P-poly(dC 12 )/RmlB and a decreasing concentration of poly(dC 12 )* were mixed with ( e ) or without ( d ) vortex. f Red fluorescence of cells harboring pBBR1MCS3a-X1 with or without l -arabinose induction. The RmlB fused with mCherry was expressed from a native promoter of rmlB in pBBR1MCS3a-X1. It caused a 2.9-fold increase in fluorescence as compared to cells harboring pBBR1MCS3. Red fluorescence was decreased 2.47-fold upon expression of rmlB asRNA from pBBR1MCS3a-X1 with 0.2% l -arabinose induction. The basal level of fluorescence with the empty vector (pBBR1MCS3) should come from the metabolites of bacteria. a.u. arbitrary units. g Persistence in cells harboring pBBR1MCS3a-X1 with or without l -arabinose induction. Expressing rmlB asRNA with 0.2% l -arabinose induction caused a nearly 24-fold decrease in persistence of the ( e ) or ( s ) cells. All experiments were performed in biological triplicates. Error bars represent standard deviations. Dot plots overlaid on bar graphs represent individual data points. Black spot, treatment step or object; arrow, treatment order Full size image We also assayed the physiological role of RmlB in persister formation. The rmlB gene is essential for viability in PAO1 since a simple knockout mutant cannot be obtained normally. Therefore, we opted for an antisense RNA (asRNA)-based approach, depleting RmlB levels by inhibiting translation of rmlB mRNA. Expression of rmlB asRNA resulted in a 2.4-fold decrease in RmlB concentration, with a nearly 24-fold decrease in persistence of the ( s ) cells, but failed to cause reduced cell growth rate (with the same doubling time of 107 min as that in a WT strain) (Fig. 2f, g ). A similar effect was also present in the corresponding ( e ) cells (Fig. 2f, g ). 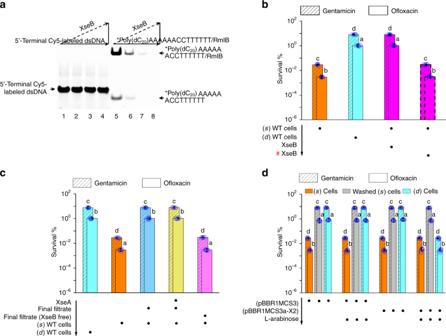Fig. 3 Extracellular XseB in-situ tailors poly(dC) at 5′ terminus.aAssays for the single strand-specific 5′ → 3′ cleavage activity of XseB. A Cy5 fluorescent label was attached to 5′ terminus of ssDNA with a hairpin structure in its 3′ terminus (5′-*poly(dC20)AAAAAACCTTTTTT-3′) or was attached to 5′ terminus of dsDNA (5′-*GTCATTCTGAGAATAGTGTAG-3′). The recombinant XseB resulted in the disappearance of fluorescence in free and RmlB-bound ssDNA rather than dsDNA.bPersistence in (s) WT cells plus recombinant XseB. The XseB-treated (s) WT cells exhibited the same persister level as that in (d) WT cells.cPersistence in (s) WT cells that was resuspended in the final filtrate plus His-tagged XseA or in the XseB-free final filtrate. Both the final filtrate and the His-tagged XseA treated final filtrate increased persistence in (s) WT cells. But the XseB-free final filtrate failed to increase persistence in (s) WT cells.dPersistence in cells expressingxseBasRNA. Plasmid pBBR1MCS3a-X2 had axseBasRNAexpression cassette. Expression ofxseBasRNAwith 0.2%l-arabinose induction caused the loss of persistence enhancement in the (d) cells. As a control, the stimulation in persistence was still present in the (d) cells harboring pBBR1MCS3a-X2 withoutl-arabinose induction. Washing increased persistence in the (s) cells harboring pBBR1MCS3a-X2 no matter with or withoutl-arabinose induction. All experiments were performed in biological triplicates. Error bars represent standard deviations. Dot plots overlaid on bar graphs represent individual data points. Black spot, treatment step or object; arrow, treatment order; hash sign, inactivated protein The MIC of antibiotics was not altered by expression of rmlB asRNA (Supplementary Table 3 ). The combined findings demonstrate that RmlB is a bona fide common binding site for both poly(dC) and P-poly(dC). Extracellular XseB in-situ switches poly(dC) to P-poly(dC) Resuspension of ( s ) WT cells (without washing) in their ( d ) supernatant led to a 10 2 - to 10 3 -fold increase in persistence (Supplementary Fig. 9a ). We subsequently observed that alkaline phosphatase treatment of the resuspended cells neutralized persistence enhancement, suggesting that the elevated persistence levels are associated with the formation of P-poly(dC)/RmlB (Supplementary Fig. 9a ). This view was confirmed following identification of P-poly(dC) as the unique RmlB-bound component in the ( d ) supernatant-treated ( s ) WT cells. Given the fact that ( s ) WT cells have possessed poly(dC)/RmlB, this result also suggests that the ( d ) WT supernatant can control in-situ switching of poly(dC) to P-poly(dC). We subsequently observed that protein activity underpinned the afore-mentioned mechanism since protease K abolished the regulatory activity of ( d ) WT supernatant during persistence (Supplementary Fig. 9b ). After ultrafiltration of the ( d ) supernatant with an Ultracel-3K Centrifugal Filter Unit (3-kDa cutoff size), the final filtrate unexpectedly enhanced persistence in ( s ) WT cells (Supplementary Fig. 9b ). This result indicates that low molecular weight protein have a critical role in the regulation of persistence. 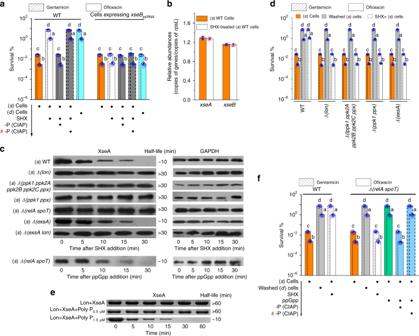Fig. 4 Involvement of stringent response in induced persistence.aPersistence in (s) WT cells plus SHX and then alkaline phosphatase (CIAP) or in (s) cells expressingxseBasRNAplus SHX. SHX increased persistence in (s) WT cells and CIAP neutralized the persistence enhancement. SHX failed to increase persistence in (s) cells expressingxseBasRNA.bQuantitative real-time PCR assays for expression ofxseBandxseAin (s) WT cells before and after plus 1 mg ml−1SHX. Copy numbers of genes were set in relation to copy numbers of housekeeping generpsL. Significant changes were not detected.cProtein involved in triggering the degradation of XseA. WT,Δ(lon),Δ(ppk1 ppk2A ppk2B ppk2C ppx), Δ(ppk1 ppx),Δ(relA spoT), Δ(exsA), andΔ(exsA lon)cells harboring pBBR1MCS3-xseA(His-tagged XseA) were grown in LB at 37 °C for 18 h ((s) phase). After addition of 1 mg ml−1SHX for 30 min, samples were removed at the indicated times for western blot analysis. (s)Δ(relA spoT)mutant harboring pBBR1MCS3-xseAwas incubated with 5 μg ml−1pp(G)pp at 37 °C for 30 min. Samples were then removed at the indicated times for western blot analysis. GAPDH was used as an internal reference.dPersistence in washed (s) mutants or SHX-treated (s) mutants. Both washing and SHX induction increased persistence in the (s)Δ(lon), (s)Δ(ppk1 ppk2A ppk2B ppk2C ppx), (s)Δ(ppk1 ppx), and (s)Δ(exsA)mutants, respectively.eSDS-PAGE analysis of in vitro degradation of XseA by Lon. His-tagged Lon failed to degrade His-tagged XseA in absence of polyP or in presence of low polyP (0.5 μM), but did it in presence of high polyP (1.5 μM).fPersistence in (s)Δ(relA spoT)mutant treated by washing, SHX induction, or ppGpp induction. Both washing and ppGpp induction increased persistence in the (s)Δ(relA spoT)mutant, but SHX induction did not. CIAP neutralized the ppGpp-triggered persistence enhancement. All experiments were performed in biological triplicates. Error bars represent standard deviations. Dot plots overlaid on bar graphs represent individual data points. Black spot, treatment step or object; arrow, treatment order; hash sign, inactivated protein Following analysis of the proteome in the final filtrate, we observed only one potential in-situ switch related protein, which has been annotated as a putative exonuclease VII small subunit XseB (8.8 kDa; locus tag, PA4042) (Supplementary Table 4 ). In the following tests, His-tagged XseB failed to degrade Cy5-labeled double-stranded DNA, but did exhibit single strand-specific 5′ → 3′ cleavage activity, which resulted in the rapid disappearance of fluorescence in both free and RmlB-bound ssDNA containing a hairpin structure in 3′ terminus and a Cy5 label (*) attached to 5′ terminus (5′-*poly(dC 20 )AAAAAACCTTTTTT-3′) (Fig. 3a ). We also observed the expected stimulation of persistence following addition of His-tagged XseB to ( s ) WT cells (Fig. 3b ). P-poly(dC) was subsequently identified as the unique RmlB-bound component in these cells. On the other hand, His-tagged XseA, a putative exonuclease VII large subunit (50.5 kDa; locus tag, PA3777), in vitro binds His-tagged XseB to form a complex that can be trapped by Ultracel-30K Centrifugal Filter Units (30-kDa cutoff size) (Supplementary Fig. 9c ). The His-tagged XseA addition did not alter the regulatory activity of persistence in the final filtrate (Fig. 3c ). Subsequently, we specifically removed XseB from the final filtrate by the trapping (Supplementary Table 4 ). The absence of XseB directly led to the loss of the regulatory activity of persistence in the filtrate (Fig. 3c ). Consistent with this, we failed to detect the free extracellular XseB along with its related stimulation in persistence in the ( d ) cells expressing xseB asRNA (Fig. 3d ; Supplementary Table 4 ) (the xseB gene is also essential for viability in PAO1 since a simple knockout mutant is not obtained). The poly(dC)/RmlB complex was not altered by the xseB asRNA since the regulatory activity in relation to persistence (i.e., washing-induced persister formation) was still present in the ( s ) cells (Fig. 3d ) (hereafter if washing stimulation in persistence was not altered, the poly(dC)/RmlB complex was determined to be unchanged). The cell growth rate and MIC of antibiotics were not altered, either. In addition, comparative proteomic analysis showed that native XseB was only present in ( d ) WT supernatant and was absent in ( e ) and ( s ) WT supernatants (Supplementary Table 4 ). All these results demonstrate that free extracellular XseB is responsible for the in-situ switch of poly(dC) to P-poly(dC). Fig. 3 Extracellular XseB in-situ tailors poly(dC) at 5′ terminus. a Assays for the single strand-specific 5′ → 3′ cleavage activity of XseB. A Cy5 fluorescent label was attached to 5′ terminus of ssDNA with a hairpin structure in its 3′ terminus (5′-*poly(dC 20 )AAAAAACCTTTTTT-3′) or was attached to 5′ terminus of dsDNA (5′-*GTCATTCTGAGAATAGTGTAG-3′). The recombinant XseB resulted in the disappearance of fluorescence in free and RmlB-bound ssDNA rather than dsDNA. b Persistence in ( s ) WT cells plus recombinant XseB. The XseB-treated ( s ) WT cells exhibited the same persister level as that in ( d ) WT cells. c Persistence in ( s ) WT cells that was resuspended in the final filtrate plus His-tagged XseA or in the XseB-free final filtrate. Both the final filtrate and the His-tagged XseA treated final filtrate increased persistence in ( s ) WT cells. But the XseB-free final filtrate failed to increase persistence in ( s ) WT cells. d Persistence in cells expressing xseB asRNA . Plasmid pBBR1MCS3a-X2 had a xseB asRNA expression cassette. Expression of xseB asRNA with 0.2% l -arabinose induction caused the loss of persistence enhancement in the ( d ) cells. As a control, the stimulation in persistence was still present in the ( d ) cells harboring pBBR1MCS3a-X2 without l -arabinose induction. Washing increased persistence in the ( s ) cells harboring pBBR1MCS3a-X2 no matter with or without l -arabinose induction. All experiments were performed in biological triplicates. Error bars represent standard deviations. Dot plots overlaid on bar graphs represent individual data points. Black spot, treatment step or object; arrow, treatment order; hash sign, inactivated protein Full size image Mechanism underlying formation of free extracellular XseB The bacterial stringent response to nutrient limitation is a key determinant in the regulation of persistence [18] , [36] , [37] . Here, the P-poly(dC)/RmlB complex that is responsible for enhanced persistence was present in the death phase, suggesting a link between complex formation and stringent response. To investigate this hypothesis, we used the amino acid starvation inducer serine hydroxamate (SHX) to trigger the stringent response in ( s ) WT cells. The resultant stimulation in persistence was neutralized following alkaline phosphatase treatment, showing that P-poly(dC)/RmlB is present in the SHX-treated ( s ) WT cells (Fig. 4a ). Free extracellular XseB was also present in these cells (Supplementary Table 4 ). Expression of xseB asRNA caused the loss of persistence phenotypic variation in the ( s ) cells following addition of SHX (Fig. 4a ). These results indicate that stringent response is dependent on XseB-mediated complex switch to induce P-poly(dC)/RmlB formation. Fig. 4 Involvement of stringent response in induced persistence. a Persistence in ( s ) WT cells plus SHX and then alkaline phosphatase (CIAP) or in ( s ) cells expressing xseB asRNA plus SHX. SHX increased persistence in ( s ) WT cells and CIAP neutralized the persistence enhancement. SHX failed to increase persistence in ( s ) cells expressing xseB asRNA . b Quantitative real-time PCR assays for expression of xseB and xseA in ( s ) WT cells before and after plus 1 mg ml −1 SHX. Copy numbers of genes were set in relation to copy numbers of housekeeping gene rpsL . Significant changes were not detected. c Protein involved in triggering the degradation of XseA. WT, Δ(lon) , Δ(ppk1 ppk2A ppk2B ppk2C ppx), Δ(ppk1 ppx) , Δ(relA spoT), Δ(exsA) , and Δ(exsA lon) cells harboring pBBR1MCS3- xseA (His-tagged XseA) were grown in LB at 37 °C for 18 h (( s ) phase). After addition of 1 mg ml −1 SHX for 30 min, samples were removed at the indicated times for western blot analysis. ( s ) Δ(relA spoT) mutant harboring pBBR1MCS3- xseA was incubated with 5 μg ml −1 pp(G)pp at 37 °C for 30 min. Samples were then removed at the indicated times for western blot analysis. GAPDH was used as an internal reference. d Persistence in washed ( s ) mutants or SHX-treated ( s ) mutants. Both washing and SHX induction increased persistence in the ( s ) Δ(lon) , ( s ) Δ(ppk1 ppk2A ppk2B ppk2C ppx) , ( s ) Δ(ppk1 ppx) , and ( s ) Δ(exsA) mutants, respectively. e SDS-PAGE analysis of in vitro degradation of XseA by Lon. His-tagged Lon failed to degrade His-tagged XseA in absence of polyP or in presence of low polyP (0.5 μM), but did it in presence of high polyP (1.5 μM). f Persistence in ( s ) Δ(relA spoT) mutant treated by washing, SHX induction, or ppGpp induction. Both washing and ppGpp induction increased persistence in the ( s ) Δ(relA spoT) mutant, but SHX induction did not. CIAP neutralized the ppGpp-triggered persistence enhancement. All experiments were performed in biological triplicates. Error bars represent standard deviations. Dot plots overlaid on bar graphs represent individual data points. Black spot, treatment step or object; arrow, treatment order; hash sign, inactivated protein Full size image Since small subunit XseB is complexed with large subunit XseA in cells, upshift of XseB expression, downshift of XseA expression, or degradation of XseA are all possible strategies to produce free XseB. SHX failed to alter the transcription of xseB and xseA but led to a rapid His-tagged XseA degradation in the ( s ) cells, indicating the presence of a separate cell-mediated strategy (Fig. 4b, c ). Previous studies have supported a role of the ubiquitous Lon protease in persister formation [18] , [32] . Given proteases are more likely to degrade XseA, we investigated the possibility of XseA as the target of Lon. As expected, His-tagged XseA was stabilized in the ( s ) Δ(lon) mutant following addition of SHX (Fig. 4c ). Consistent with this, free extracellular XseB along with its related stimulation in persistence was not present in the SHX-treated ( s ) Δ(lon) mutant (Fig. 4d ; Supplementary Table 4 ). The cell doubling time (107 min) and poly(dC)/RmlB were not altered by deletion of lon (Fig. 4d ). Interestingly, we did not observe the His-tagged Lon-mediated His-tagged XseA degradation in vitro even if the former was excessive (Fig. 4e ). Given in E. coli , polyP, the only known Lon-activator, combines with and stimulates Lon to degrade the ribosomal protein in response to starvation [38] , it would appear that polyP is required for Lon degradation of XseA in PAO1. To investigate this hypothesis, we deleted four known polyphosphate kinase ( ppk ) genes including ppk1 (PA5242), ppk2A (PA0141), ppk2B (PA2428), and ppk2C (PA3455)) and one known polyphosphate exopolyphosphatase ( ppx ) gene (PA5241) in PAO1. The deletions did not affect the cell doubling time (107 min) and poly(dC)/RmlB (Fig. 4d ). The resultant mutant remained a low level of polyP (0.48 μM) in its ( s ) cells following addition of SHX. A similar effect was also observed in the Δ(ppk1 ppx) mutant (Fig. 4d ). In contrast, the WT strain markedly elevated polyP level from 0.32 to 4.4 μM in its ( s ) cells upon SHX treatment. We then observed the stable His-tagged XseA in both ( s ) mutants following addition of SHX (Fig. 4c ). This may account for the subsequent loss of free extracellular XseB along with its related stimulation in persistence (Fig. 4d ; Supplementary Table 4 ). In vitro, His-tagged XseA still remained stable even after 60 min in presence of 0.5 μM polyP, but was rapidly degraded by His-tagged Lon in presence of 1.5 μM polyP (Fig. 4e ). These results indicate a close linkage between the stringent response, polyP accumulation and Lon-mediated XseA degradation. Alarmone (p)ppGpp is the ubiquitous regulator of stringent response. Deletion of (p)ppGpp synthetase genes relA and spot can interrupt the stringent response. This led to a low polyP level (0.37 μM) and a stable His-tagged XseA along with the loss of free extracellular XseB and persistence enhancement in the ( s ) Δ(relA spoT) mutant following addition of SHX (Fig. 4c, f ; Supplementary Table 4 ). The cell doubling time (107 min) and poly(dC)/RmlB were not altered by the deletions (Fig. 4f ). The chemical ppGpp recovered the stringent response in this ( s ) mutant, thereby promoting polyP accumulation to 3.8 μM and His-tagged XseA degradation, ultimately resulting in free extracellular XseB and its related persistence stimulation that was neutralized following dephosphorylation (Fig. 4c, f ; Supplementary Table 4 ). These indicate that the stringent response is dependent on (p)ppGpp to promote polyP accumulation. XseB lacks an amino-terminal signal peptide. Consequently, the translocation of this protein may require a Sec-independent secretion system. Previous studies have suggested a close link between P. aeruginosa persistence and the Sec-independent T3SS since overexpression of HigB upshifts T3SS expression while knockout of relA and spot genes downshifts T3SS expression [31] , [39] . We then investigated whether T3SS is responsible for the extracellular secretion of XseB. The Δ(exsA) mutant is defective for expression and secretion of T3SS-related exoproducts [40] . It is also defective in delivery of XseB since the extracellular XseB along with its related stimulation in persistence was not observed in the ( s ) Δ(exsA) mutant following addition of SHX (Fig. 4d ; Supplementary Table 4 ). Deletion of exsA did not affect the cell doubling time (107 min) and poly(dC)/RmlB (Fig. 4d ). Nor did it alter the Lon-mediated XseA/XseB dissociation because the rapid Hig-tagged XseA degradation was still present in the ( s ) Δ(exsA) mutant following addition of SHX; conversely, it was absent in the SHX-treated ( s ) Δ(exsA lon) mutant (Fig. 4c ). Thus, in summary these data reveal a (p)ppGpp-controlled signaling pathway that contains polyP, Lon, exonuclease VII (XseA/XseB), and T3SS. Complex switch mediates persistence through reduction of PMF The switching of poly(dC)/RmlB to P-poly(dC)/RmlB (by afore-mentioned His-tagged XseB or a T4 polynucleotide kinase-mediated poly(dC) in-situ phosphorylation) or to DNA-free RmlB (by washing) could directly induce persistence in PAO1 without the requirement for other protein since elevated levels of persistence were present in the protein synthesis-blocked ( s ) WT cells (Supplementary Fig. 10a ). RmlB is located on cell membrane, to which the proton gradient-dependent energy-generating machinery is tightly coupled. Previous studies have shown that hydrophobic GhoT, HokB, and TisB peptides can dissipate PMF across the membrane thereby reducing intracellular ATP levels by compromising cell membrane integrity. The resultant considerable energy loss directly reduces multiple cellular metabolic processes, thereby leading to persistence [15] , [41] , [42] , [43] , [44] . Thus, we next investigated whether the complex switch independently affected the PMF and intracellular ATP levels. Potential-sensitive dye DiBAC 4 (3) and a luciferase-based assay were used to assess changes in PMF and intracellular ATP concentration, respectively [42] , [43] , [44] . The RFP label was used to visualize cells. Treatment of ( s ) WT cells with His-tagged XseB or T4 polynucleotide kinase resulted in a marked reduction in PMF and a nearly 80-fold reduction in cellular ATP levels (Fig. 5a, b ). Subsequent dephosphorylation ameliorated both of these effects (Fig. 5c, d ). Washing of ( s ) WT cells led to a similar decrease in PMF and cellular ATP levels (nearly 77-fold) (Supplementary Fig. 10b, c ). And post-treatment with poly(dC 12 ) instead of P-poly(dC 12 ) eliminated these negative effects (Supplementary Fig. 10b, c ). In addition, in-situ phosphorylation resulted in a sharp reduction in PMF and cellular ATP levels in poly(dC 12 )-pretreated washed ( s ) WT cells (Supplementary Fig. 10d, e ). Instead, in-situ dephosphorylation led to a marked increase in PMF and cellular ATP levels in P-poly(dC 12 )-pretreated washed ( s ) WT cells (Supplementary Fig. 10f, g ). These results indicated that cells could decrease PMF and intracellular ATP levels in response to poly(dC) removal or in-situ complex switching. The resultant high levels of persistence might be considered an adaptive response to the reduction in intracellular energy. Furthermore, we consistently observed a reduction in PMF and lower cellular ATP levels in ( d ) WT cells (Fig. 5e, f ). To further investigate this phenomenon, we utilized d -mannitol to promote PMF in ( d ) WT cells [44] , [45] . As expected, d -mannitol abolished the effect of P-poly(dC)/RmlB on PMF and cellular ATP levels as well as persistence (Fig. 5e , f; Supplementary Fig. 10h ). Fig. 5 PMF and intracellular ATP levels during complex switching. a , b PMF and intracellular ATP levels of ( s ) WT cells plus recombinant XseB or T4 polynucleotide kinase. c , d PMF and intracellular ATP levels of XseB-treated ( s ) WT cells or T4 polynucleotide kinase-treated ( s ) WT cells, both of which were treated with CIAP. Addition of CIAP did not affect PMF of ( s ) WT cells. e , f PMF and intracellular ATP levels of ( s ) WT cells, ( d ) WT cells, or ( d ) WT cells plus d -mannitol. All experiments were performed in biological triplicates. Error bars represent standard deviations. Dot plots overlaid on bar graphs represent individual data points. Black spot, treatment step or object; arrow, treatment order; hash sign, inactivated protein Full size image Persistence might be a response to rhamnose pathway shutdown Four contiguous genes ( rmlBDAC ) in PAO1 have been reported to be responsible for the biosynthesis of dTDP- l -rhamnose [46] . RmlB has previously been assigned as a putative dTDP- d -glucose 4,6-dehydratase. An RmlB homolog (RmlB′, sharing 61% identity) in E. coli K-12 can catalyze the dehydration of dTDP- d -glucose to dTDP-4-keto-6-deoxy- d -glucose [47] ; however RmlB (expressed in E. coli ) itself is incapable of catalyzing the same reaction (Supplementary Fig. 11a ). Given native RmlB is present in PAO1 as poly(dC)/RmlB or P-poly(dC)/RmlB, we decided to assay the in vitro catalytic activities of poly(dC 12 )/RmlB and P-poly(dC 12 )/RmlB. Interestingly, the former promoted dehydration whereas the latter did not (Supplementary Fig. 11a ). This result indicated that poly(dC)/RmlB functions as a bona fide dTDP- d -glucose 4,6-dehydratase. Thus, it is more likely that in vivo switching of poly(dC)/RmlB to P-poly(dC)/RmlB or RmlB results in the same loss in dehydration activity, thereby shutting down the dTDP- l -rhamnose pathway. The hypothesis was supported by the observation that a sharp reduction in intracellular free rhamnose concentration was present within 20 min after treatment of ( s ) WT cells with His-tagged XseB (from 64.9 to 8.2 mg l −1 ) or washing step (from 64.9 to 10.4 mg l −1 ). The reduction was not associated with the complex switch-triggered cellular PMF decrease since the high rhamnose level (63.6 mg l −1 ) was still present in ( s ) WT cells treated even for 2 h with the proton ionophore carbonyl cyanide m-chlorophenyl hydrazone (CCCP), which decreases PMF directly [45] . On the other hand, the rmlB gene is essential for viability in PAO1 since the Δ(rmlB) mutant is unable to survive in LB medium (Supplementary Fig. 11b ). It is likely that the RmlB-mediated dormancy mechanism underpins this phenomenon. Furthermore, we also found that deletion of other rml genes ( Δ(rmlA) , Δ(rmlC) , and Δ(rmlD) ) also resulted in growth inhibition (Supplementary Fig. 11b ). Conversely, all of these mutants were capable of surviving in LB plus rhamnose (Supplementary Fig. 11b ). Our results also revealed that the dTDP- l -rhamnose pathway is essential for PAO1 viability. It is likely that shutdown of this pathway inhibits cell wall synthesis since rhamnose is a fundamental component of the PAO1 cell wall [48] . Switching of poly(dC)/RmlB to P-poly(dC)/RmlB or RmlB results in similar phenomena as knockout of rmlB , with a concomitant reduction in dehydration activity and shutdown of the dTDP- l -rhamnose pathway. These occurrences can cause lethality in associated cells. Thus, the complex switch-triggered persistence might be considered as an adaptive response to the adverse conditions. In this study, we revealed a microbial strategy for the rapid regulation of P. aeruginosa PAO1 persistence. This strategy is based on switching of the membrane-associated complex poly(dC)/RmlB to P-poly(dC)/RmlB by extracellular XseB-mediated in-situ tailoring of poly(dC) to P-poly(dC) (Fig. 6 ). In response to the switch, bacteria dissipate cell membrane PMF and reduce intracellular ATP levels with generation of a concomitant increase in persistence. Switching of the complex is linked to an alarmone (p)ppGpp-controlled signaling pathway in which (p)ppGpp, polyP accumulation, and Lon-mediated intracellular exonuclease VII large subunit XseA degradation were invoked; the free exonuclease VII small subunit XseB is transported to extracellular space by T3SS where it exhibits 5′ → 3′ cleavage activity on RmlB-bound poly(dC). This reaction results in in-situ switching of poly(dC)/RmlB to P-poly(dC)/RmlB. Alternatively, in-situ phosphorylation or appropriate washing of PAO1 causes direct switching of poly(dC)/RmlB to P-poly(dC)/RmlB or DNA-free RmlB without the requirement for the (p)ppGpp-controlled signaling pathway. In response to both approaches, bacteria reduce cellular PMF and ATP levels. Finally, in this study we report that poly(dC)/RmlB functions as a dTDP- d -glucose 4,6-dehydratase in the dTDP- l -rhamnose pathway. Switching of poly(dC)/RmlB to P-poly(dC)/RmlB or RmlB causes a reduction in catalytic activity loss, thereby leading to the shutdown of the dTDP- l -rhamnose pathway. This shutdown is lethal. Thus the complex switch-triggered persistence also might be an adaptive response to the pathway shutdown. Fig. 6 A proposed model explaining poly(dC)/RmlB-mediated persistence. Activation of RelA or SpoT induces a (p)ppGpp-controlled signaling pathway, which invokes Lon to degrade intracellular exonuclease VII large subunit XseA. Free exonuclease VII small subunit XseB is delivered to extracellular space by T3SS and tailors RmlB-bound poly(dC) to form P-poly(dC), which results in in-situ switch of poly(dC)/RmlB to P-poly(dC)/RmlB. On the other hand, in-situ phosphorylation or washing of PAO1 can bypass the (p)ppGpp-controlled signaling pathway and directly switch poly(dC)/RmlB to P-poly(dC)/RmlB or individual RmlB. In response to the switch in the complex physiological state, cells decrease PMF and intracellular ATP level and shutdown the dTDP- l -rhamnose pathway, forming persistence in PAO1 Full size image RmlB is a ubiquitous protein in microorganisms. RmlB in PAO1 shares high identity (>70%) with its homologs in other Pseudomonas spp. We do not know whether poly(dC) is ubiquitous in these strains, but the RmlB sequence suggests that they share a cognate RmlB-based persister formation mechanism with PAO1. Furthermore, the sequence similarity indicates that washing or in-situ phosphorylation might lead to an apparent increase in the persistence of these species. This hypothesis was initially supported by the observation of a 10 2 - to 10 3 -fold increase in persistence of stationary phase P. aeruginosa (ATCC 9027) (a clinical isolate), P. putida KT2440, P. mendocina (ATCC 25411), P. chlororaphis (ATCC 9446), P. stutzeri (CICC 10402), P. fluorescens (CICC 21093), and P. maltophilia (CICC 20702) cells in response to washing or in-situ phosphorylation (Supplementary Fig. 12 ). To further investigate the phenomenon, we measured the persistence in death phase of each bacteria. As expected, all of the strains exhibited a reversible persistence enhancement that was neutralized following alkaline phosphatase treatment (dephosphorylation) (Supplementary Fig. 12 ). The presence of a cognate regulatory strategy in different species demonstrates the ubiquitous nature of this approach in the Pseudomonas genus. Of note, RmlB in PAO1 shares a high identity (61%) with its homolog RmlB′ in E. coli K-12. However, we did not observe an increased persistence phenotype after washing or in-situ phosphorylation of stationary phase E. coli K-12 cells (Supplementary Fig. 13a ). This regulation failure was also observed in stationary phase Rhodococcus jostii RHA1, Bacillus amyloliquefaciens SQR9, and Streptococcus thermophilus ND03 cells, where associated RmlB homologs share reduced identity (less than 50%) with the PAO1 protein (Supplementary Fig. 13b-d ). These results indicate an absence of RmlB-based regulatory strategies in other genus strains, implying its uniqueness in Pseudomonas and raising the possibility that RmlB evolution lines are different between Pseudomonas spp. and other bacteria. Many questions still remain unanswered concerning how and where the poly(dC) is generated. Several poly(dC) molecules are longer than 9 bases, but the corresponding dC strings (>9 bases) are not present in PAO1 genome, suggesting that all poly(dC) are not the direct derivatives from the genome. Thus, we speculated that poly(dC) might be synthesized. We exploited the random insertional mutagenesis to screen for bacterial genes responsible for poly(dC) synthesis. The target mutant with the integral rmlB gene should either lose the washing stimulation in persistence or be unable to survive unless addition of poly(dC). However, none of tested mutants exhibited the phenotypes. It is possible that poly(dC) generation is controlled by some overlapping mechanisms involving different gene families in a cooperative manner. In addition, we found poly(dC) in extracellular space. It is likely that poly(dC) is synthesized in the space. However, this hypothesis seemed not to be supported by the observation that extracellular protein extracts failed to elongate the length of poly(dC 4 ) with a Cy5 label (*) attached to its 5′ terminus following addition of dCTP (Supplementary Fig. 14a ). Puzzlingly, it seems impossible for poly(dC) to be synthesized within cells since ( e ) and ( s ) intracellular total DNA extracts did not reduce persistence in washed ( e ) WT cells and washed ( s ) WT cells, respectively (Supplementary Fig. 14b ). Thus, at present the location of poly(dC) synthesis still remains unknown. Nor did it be determined whom the synthesis is initiated with. The origin of poly(dC) requires further investigation. Protein phosphorylation is a ubiquitous post-translational modification in all three kingdoms of life. It has a crucial role in the regulation of all kinds of physiological processes and mediates rapid and efficient bacterial responses and adaptation mechanisms to hostile environments [49] . Although XseB exerts a single strand-specific 5′ → 3′ tailor function in this study, the XseB-mediated complex switch (poly(dC)/RmlB to P-poly(dC)/RmlB) can be considered as a non-typical protein phosphorylation event since the phosphate group modifies the complex function. Furthermore, the modification is very different from almost all known protein phosphorylation events. For example, compared to most common types of bacterial protein phosphorylation events (namely on serine, threonine, tyrosine, histidine, or aspartate residues) [49] , the phosphate group is present on a nucleotide instead of an amino acid residue. In addition, its formation is dependent on exonuclease VII small subunit XseB rather than a versatile repertoire of protein kinases or phosphatases. XseB-mediated incomplete degradation of RmlB-bound poly(dC) has a pseudo-phosphorylation role on DNA as well as on the complex itself. Typical protein phosphorylation events regulate protein function while causing alterations to the structural conformation of substrates. DNA pseudo-phosphorylation also regulates poly(dC)/RmlB function, suggesting that this pseudo-phosphorylation event might induce a conformational change in RmlB or RmlB complexes. In addition, this pseudo-phosphorylation also suggests that bacterial protein phosphorylation events may be far more variable in outcome than those previously encountered. Furthermore, the phosphorylation site is obviously not limited to amino acid residues in bacterial cells. Unfortunately, we do not know at present why bacteria utilize pseudo-phosphorylation rather than bona fide protein phosphorylation to regulate complex function. Perhaps this represents a novel evolutionary diversification strategy. Switching of P-poly(C)/RmlB back to its unphosphorylated state causes a marked reduction (10 2 - to 10 3 -fold) in persistence of a ( d ) WT PAO1 cells, suggesting a potential persister wake-up mechanism (Supplementary Fig. 7g, h ). The residual reduction in the levels of persistence indicates the presence of alternative mechanisms (perhaps TA modules) that elicit this phenotype. Besides the (p)ppGpp-controlled signaling pathway, switching of poly(dC)/RmlB can also be triggered by extracellular DNA cleavage or phosphorylation. We believe that these findings will help us to further understand the phenomenon of multidrug resistance in clinical P. aeruginosa isolates. Factually, the clinical isolate P. aeruginosa (ATCC 9027) did also exhibit the RmlB-based persister formation (Supplementary Fig. 12b ). It is likely that bacteria rapidly increase persistence by means of environmental nucleases, phosphatases, or protein kinases, thereby showing a phenotypic tolerance to clinical antibiotics. General methods Full methods are available in the Supplemental Experimental Procedures. Bacterial strains Parent strains including P. aeruginosa PAO1, P. aeruginosa (ATCC 9027), P. putida KT2440, P. stutzeri (CICC 10402), P. fluorescens (CICC 21093), E. coli K-12 MG1655, and Bacillus amyloliquefaciens SQR9, RFP-labeled P. aeruginosa PAO1 strain (harboring plasmid pYC12- mCherry ), most of P. aeruginosa PAO1 mutants, and tool strains including E. coli DH5α, E. coli BL21 (DE3) pLysS, and E. coli SM10 ( λ pir ) were all grown at 37 °C in Luria-Bertani (LB) medium (pH 7.2). Parent strains including P. mendocina (ATCC 25411), P. chlororaphis (ATCC 9446), P. maltophilia (CICC 20702), Rhodococcus jostii RHA1, and Streptococcus thermophilus ND03 were grown at 30 °C in LB medium. P. aeruginosa PAO1 mutants including Δ(rmlA) , Δ(rmlB) , Δ(rmlC) , and Δ(rmlD) were grown at 37 °C in LB plus 1 mg ml −1 rhamnose. Plasmid pYC12- mCherry was a kind gift from Pro. Yangchun Xu (Jiangsu Provincial Key Lab of Organic Solid Waste Utilization, Nanjing Agricultural University). Minimum inhibitory concentration (MIC) MICs of ofloxacin and gentamicin were determined for all bacterial strains used in this study as described previously [34] , [44] . Bacterial colonies were incubated with 250 rpm in liquid LB to exponential, stationary, or death phase and treated with or without each potential persistence effector for 1 h. The pH of medium was not altered by these effectors. Cells were then diluted to 10 5 CFU ml −1 in liquid LB plus 0.025 to 3.0 μg ml −1 ofloxacin or 0.1 to 50 μg ml −1 gentamicin, and incubated with 250 rpm for at least 30 h. OD 600 was measured at inoculation and after 30-h incubation to determine growth. Supplementary Table 3 listed MICs. The addition of each effector did not alter bacterial MICs. For persistence assays, antibiotic treatments were ≥ 10 × MIC to ensure killing of sensitive cells. Standard persistence assays Bacterial colonies were incubated in LB to stationary phase. Cells were then diluted to 10 5 CFU ml −1 in LB and grown with 250 rpm to different phase. Cells were plated for CFU counts and then diluted to 10 5 CFU ml −1 in liquid LB for antibiotic challenge. For P. aeruginosa PAO1, 10 μg ml −1 ofloxacin or 50 μg ml −1 gentamicin was used in an assay [34] . For E. coli K-12, 5 μg ml −1 ofloxacin or 20 μg ml −1 gentamicin was used in an assay [44] . For other bacteria, ofloxacin and gentamicin concentrations were listed in Supplementary Table 3 . At each timepoint, an aliquot of cells was removed, washed with 0.75% NaCl and plated to enumerate survivors. In this study, all challenges were performed for 3 h because each antibiotic treatment eliminated all susceptible non-persister cells. There was no significant growth differences between P. aeruginosa PAO1 (WT) and its mutants as well as both PTasRNA-expressing strains in this study. Thus, we named their exponential (i.e., 6 h), stationary (i.e., 18 h), and death phase (i.e., 39 h) as ( e ), ( s ), and ( d ), respectively. Other stationary phase bacteria referred to P. aeruginosa (ATCC 9027) (16-h), P. putida KT2440 (16-h), P. mendocina (ATCC 25411) (16-h), P. chlororaphis (ATCC 9446) (16-h), P. stutzeri (CICC 10402) (16-h), P. fluorescens (CICC 21093) (16-h), P. maltophilia (CICC 20702) (8-h), E. coli K-12 (16-h), Rhodococcus jostii RHA1 (30-h), Bacillus amyloliquefaciens SQR9 (30-h), and Streptococcus thermophilus ND03 (30-h). Other death phase bacteria referred to P. aeruginosa (ATCC 9027) (42-h), P. putida KT2440 (42-h), P. mendocina (ATCC 25411) (42-h), P. chlororaphis (ATCC 9446) (42-h), P. stutzeri (CICC 10402) (42-h), P. fluorescens (CICC 21093) (42-h), and P. maltophilia (CICC 20702) (26-h). Treatment of cells prior to antibiotic challenges The specific objects of “cells” or “washed cells” were referred in the main text. Several treatments were combined to use in some experiments. Centrifugation: Cells were centrifuged at 12,000 × g for 3 min at room temperature and resuspended in an equal volume of spent LB. Washing: Cells were washed three times by sterile water using a vortex meter and resuspended in an equal volume of fresh LB medium (unless otherwise stated) without pH alternation (even plus potential persistence effector). An aliquot of washed cells was diluted to 10 5 CFU ml −1 in LB and grown with 250 rpm. OD 600 was measured periodically to determine the regrowth curve. Chemicals: Cells or washed cells were incubated with 1 mg ml −1 SHX, 5 μg ml −1 pp(G)pp, 100 μg ml −1 gentamicin (as the protein synthesis blocker), 10 mM mannitol, or 100 mg l −1 extracellular chemical extracts at 37 °C for 30 min. The extracellular chemical extracts were prepared by extraction of supernatant with ethyl acetate three times and chloroform twice. The extracts were dissolved in DMSO. Supernatants: Washed cells were resuspended in proteinase K-, RNase A-, DNase I-, exonuclease I-, or exonuclease III-treated supernatant at room temperature for 10 min. Cells were resuspended in XseB-free supernatant at room temperature for 10 min. Each enzyme treatment was performed at 37 °C for 2 h. Proteinase K, DNase I, exonuclease I, and exonuclease III were heat-inactivated at 95 °C for 15 min. RNase A was inactivated by 0.1% DEPC. The XseB-free supernatant was prepared as follows: His-tagged XseA was incubated with supernatant at 37 °C for 30 min; the formed XseA/XseB complex was trapped by an Ultracel-3K Centrifugal Filter Unit (3-kDa cutoff size). The filtrate was the XseB-free supernatant. Extracellular ssDNA: Washed cells were resuspended in DNA-free supernatant plus 0.1 μg ml −1 extracellular ssDNA or its phosphorylated product at room temperature for 10 min. The ssDNA extraction and phosphorylation were as follows: proteinase K and RNase A were used to remove protein and RNA from a filter-sterilized supernatant; the treated supernatant was ultrafiltered to remove dsDNA and residual protein by Amicon Ultracel-3K Centrifugal Filter Units; exonuclease III was finally used to remove residual dsDNA from the filtrate. Extracellular ssDNA was then extracted and dissolved in water at 20 ng μl −1 . An aliquot of ssDNA was phosphorylated by incubation with T4 polynucleotide kinase at 37 °C for 1 h. The DNA-free supernatant was prepared by incubation of filter-sterilized supernatant with DNase I that was then heat-inactivated. Poly(dC), P-poly(dC), or other ssDNA: Cells or washed cells were usually incubated with poly(dC), P-poly(dC), poly(dC) mutants, poly(dC) derivatives, P-poly(dC) derivative, poly(dC)/P-poly(dC) or other ssDNAs at a final concentration of 10 μM at room temperature for 10 min. For assay of dose-effect relation between poly(dC) and persistence, washed ( e ) WT cells or washed ( s ) WT cells were incubated with poly(dC) at a final concentration from 10 to 10 −6 μM at room temperature for 10 min. Poly(dC) included poly(dC 6,8,9,12,20,30,40 ) and P-poly(dC) included P-poly(dC 6,8,9,12,20,30,40 ). 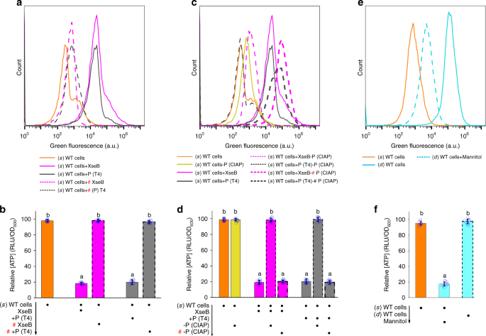Fig. 5 PMF and intracellular ATP levels during complex switching.a,bPMF and intracellular ATP levels of (s) WT cells plus recombinant XseB or T4 polynucleotide kinase.c,dPMF and intracellular ATP levels of XseB-treated (s) WT cells or T4 polynucleotide kinase-treated (s) WT cells, both of which were treated with CIAP. Addition of CIAP did not affect PMF of (s) WT cells.e,fPMF and intracellular ATP levels of (s) WT cells, (d) WT cells, or (d) WT cells plusd-mannitol. All experiments were performed in biological triplicates. Error bars represent standard deviations. Dot plots overlaid on bar graphs represent individual data points. Black spot, treatment step or object; arrow, treatment order; hash sign, inactivated protein Poly(dC) mutants were listed in Supplementary Table 5 . Poly(dC) derivatives included exonuclease I-partially digested poly(dC 12 ), DNase I-partially digested poly(dC 12 ), and poly(dC 12 )*. P-poly(dC) derivative included P-poly(dC 12 )*. Poly(dC 12 ) and P-poly(dC 6,12,30 ) were used to form the mixture. The molar ratios of poly(dC 12 ) and each P-poly(dC) were 1:1, 1:10 −1 , 1:10 −2 , 1:10 −3 , and 1:10 −4 , respectively. Poly(dC 12 ) and P-poly(dC 12 )* were used to form the mixture at the molar ratio of 1:1. Other ssDNAs included ATG TGC AGT C*, P-ATG TGC AGT C*, CCG TTG CAT GCC GTA CGC GA*, P-CCG TTG CAT GCC GTA CGC GA*, TGT CTA AGT CAG TAA CTT GAC TGA CCG TGC*, and P-TGT CTA AGT CAG TAA CTT GAC TGA CCG TGC*. Enzymes: Cells or washed cells were incubated with alkaline phosphatase (calf intestine) at 37 °C for 30 min, T4 polynucleotide kinase at 37 °C for 1 h, 10 μg ml −1 trapped protein (by ultrafiltration) at room temperature for 10 min, or 10 μg ml −1 His-tagged XseB at room temperature for 10 min. Each inactivated enzyme was also used as a control. Alkaline phosphatase (calf intestine), T4 polynucleotide kinase, and His-tagged XseB were heat-inactivated at 95 °C for 1 h, respectively. Intracellular total DNA: Washed cells were incubated with 0.1 μg ml −1 intracellular total DNA extracts at room temperature for 10 min. Preparation of membrane protein After formaldehyde cross-linkage, cells were resuspended in PBS and disrupted by sonication. After centrifugation at 3000 × g for 5 min at 4 °C, the supernatant was collected, and then centrifuged at 15,000 × g , 4 °C for 30 min. The membrane and membrane protein were washed twice. The membrane protein were further extracted by using ProteoPrep Membrane Extraction Kit and quantified by the protein assay kit with bovine serum albumin as a standard. Extra/intracellular protein pr e paration and proteolysis Cultures were centrifuged at 12,000 × g for 5 min at room temperature. The supernatant was filter sterilized by 0.22 μm PTFE filter and ultrafiltered by Ultracel-3K Centrifugal Filter Units (3-kDa cutoff size). The filtrate was collected and freeze-dried to obtain the extracellular protein. Cells were resuspended in 10 mM Tris–HCl buffer (pH 7.5) and disrupted by sonication. After centrifugation at 15,000 × g , 4 °C for 30 min, the supernatant was collected and freeze-dried to obtain the intracellular protein. All protein were further treated by 5% stacking gel of SDS-PAGE (without running gel) subsequently. The gel was stained with silver nitrate for detection of the protein band (the stacked extracellular protein). Ingel digestion and peptide purification were performed as described above. EMSA All samples were separated by 15% native-PAGE in the experiments. All gels were scanned by Typhoon Trio-Variable Mode Imager (GE Healthcare) under the excitation of 650 nm for detection of fluorescent-labeled DNA. Activity of RmlB binding ssDNA: 0.15 mM poly(dC 12 )* or P-poly(dC 12 )* was incubated with His-tagged RmlB in 10 mM Tris–HCl buffer (pH 7.5) at room temperature for 10 min. The concentration of protein was 0, 1, 5, or 10 μg ml −1 . As controls, 10 μg ml −1 BSA was incubated with 0.15 mM poly(dC 12 )* or P-poly(dC 12 )*; 10 μg ml −1 His-tagged RmlB was incubated with each 0.15 mM ssDNA* or 0.15 mM P-ssDNA*. Order of RmlB binding poly(dC) and P-poly(dC): Poly(dC 12 )*/P-poly(dC 30 )* (0.15 mM of each) or P-poly(dC 12 )*/poly(dC 30 )* (0.15 mM of each) mixture was incubated with His-tagged RmlB in 10 mM Tris–HCl buffer (pH 7.5) at room temperature for 10 min. The concentration of protein was 0, 1, 5, 10, 15, or 20 μg ml −1 . Substitutability of RmlB-bound poly(dC): Poly(dC)/RmlB was prepared by incubation of 0.15 mM poly(dC 12 ) (excessive) with 5 μg ml −1 His-tagged RmlB in 10 mM Tris–HCl buffer (pH 7.5) at room temperature for 10 min. After centrifugation at 12,000 × g for 5 min, insoluble poly(dC)/RmlB was collected and washed twice to remove unbound poly(dC 12 ) (without violent stir). 5 μg ml −1 poly(dC)/RmlB was incubated with P-poly(dC 12 )* in 10 mM Tris–HCl buffer (pH 7.5) at room temperature for 10 min with or without vortex. The concentration of P-poly(dC 12 )* was 0.15, 0.015, or 0.0015 mM. Substitutability of RmlB-bound P-poly(dC): P-poly(dC)/RmlB was prepared by incubation of 0.15 mM P-poly(dC 12 ) (excessive) with 5 μg ml −1 His-tagged RmlB in 10 mM Tris–HCl buffer (pH 7.5) at room temperature for 10 min. After centrifugation at 12,000 × g for 5 min, insoluble P-poly(dC)/RmlB was collected and washed twice to remove unbound P-poly(dC 12 ) (without violent stir). 5 μg ml −1 P-poly(dC)/RmlB was incubated with poly(dC 12 )* in 10 mM Tris–HCl buffer (pH 7.5) at room temperature for 10 min with or without vortex. The concentration of poly(dC 12 )* was 0.15, 0.015, or 0.0015 mM. Activity of XseB cleaving dsDNA: A Cy5 fluorescent label was attached to 5′ terminus of dsDNA (5′-*GTCATTCTGAGAATAGTGTAG-3′). 0.15 mM dsDNA was incubated with His-tagged XseB in 10 mM Tris–HCl buffer (pH 7.5) at room temperature for 10 min. The concentration of protein was 0, 1, 5, or 10 μg ml −1 . Activity of XseB cleaving ssDNA from 5′ terminus: A Cy5 fluorescent label was attached to 5′ terminus of ssDNA with a hairpin structure in its 3′ terminus (5′-*poly(dC 20 )AAAAAACCTTTTTT-3′). ssDNA/RmlB was prepared by incubation of 0.15 mM *ssDNA (excessive) with 5 μg ml −1 His-tagged RmlB in 10 mM Tris–HCl buffer (pH 7.5) at room temperature for 10 min. The mixture was then incubated with His-tagged XseB at room temperature for 10 min. The concentration of His-tagged XseB was 0, 1, 5, or 10 μg ml −1 . Activity of extracellular protein in vitro synthesizing poly (dC): A Cy5 fluorescent label was attached to 5′ terminus of poly(dC 4 ). 0.15 mM *poly(dC 4 ) was incubated with extracellular protein extracts in 10 mM Tris–HCl buffer (pH 7.5) plus 0.2 mM dCTP at room temperature for 30 min. The concentration of extracellular protein extracts was 0, 1, 5, or 10 μg ml −1 . Trapping XseB in vitro 5 μg ml −1 His-tagged XseB was incubated with 100 μg ml −1 His-tagged XseA (excessive) in 10 mM Tris–HCl buffer (pH 7.5) at 37 °C for 20 min. The mixture was ultrafiltered by Amicon Ultracel-30K Centrifugal Filter Units. The filtrate and the trapped protein were then analyzed by SDS-PAGE. Induction of asRNA expression P. aeruginosa PAO1 (WT) harboring pBBR1MCS3a-X1 or pBBR1MCS3a-X2 was diluted to 10 5 CFU ml −1 in LB plus 50 μg ml −1 tetracycline. The cells were then incubated with or without 0.2% of l -arabinose at 37 °C with 250 rpm to different phase. l -arabinose was used to induce expression of each asRNA expression cassette. Red fluorescence (emitted by RFP) of samples was recorded by a BD Accuri C6 Flow Cytometer equipped with a 580 nm (red) laser and 610 nm filter. In vitro degradation activity of His-tagged Lon 0.25 or 2.5 μg μl −1 His-tagged Lon was incubated with polyP in 50 mM Tris–HCl buffer (pH 8.0) plus 7.5 mM MgCl 2 , 4 mM ATP, and 2.0 μg μl −1 His-tagged XseA at 37 °C for 60 min. The concentration of polyP was 0, 0.5 or 1.5 μM. The mixture was then analyzed by SDS-PAGE at 0, 5, 10, 15, 30, and 60 min of incubation. All uncropped scans of SDS-PAGE were shown in Supplementary Fig. 15 . Western blot analysis ( s ) WT or each ( s ) mutant was incubated with 1 mg ml −1 SHX at 37 °C for induction of amino acid starvation. ( s ) Δ(relA spoT) mutant was incubated with 5 μg ml −1 pp(G)pp at 37 °C for recovery of the stringent response. Cells were collected at 0, 5, 10, 15, and 30 min of incubation. The total protein were separated by SDS-PAGE and transferred onto a PVDF membrane and incubated with a monoclonal mouse His-tag antibody (1:2000) (Abcam, Cat#: ab5000) at 4 °C overnight. After washing with PBS plus 0.05% Tween-20 for four times, the membranes were incubated with a polyclonal horseradish peroxidase-conjugated goat anti-mouse IgG (1:2000) (Abcam, Cat#: ab85760) at 37 °C for 1 h. Signals were detected with the Optiblot ECL Detect Kit (Abcam) and visualized with a Bio-Rad molecular imager ChemiDoc MP. GAPDH was used as an internal reference. All uncropped scans of western blots were shown in Supplementary Fig. 16 . PolyP quantification Cells were washed twice with 0.9% NaCl and diluted to an OD 600 of 0.2 in water. After incubation with 10 μM 4′,6′-diamidino-2-phenylindole (DAPI) at room temperature for 20 min in the dark, the fluorescence of samples was recorded in a fluorimeter with excitation at 415 nm and emission at 550 nm. 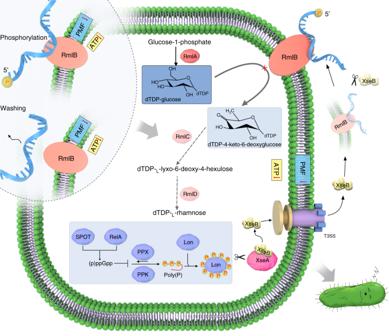Fig. 6 A proposed model explaining poly(dC)/RmlB-mediated persistence. Activation of RelA or SpoT induces a (p)ppGpp-controlled signaling pathway, which invokes Lon to degrade intracellular exonuclease VII large subunit XseA. Free exonuclease VII small subunit XseB is delivered to extracellular space by T3SS and tailors RmlB-bound poly(dC) to form P-poly(dC), which results in in-situ switch of poly(dC)/RmlB to P-poly(dC)/RmlB. On the other hand, in-situ phosphorylation or washing of PAO1 can bypass the (p)ppGpp-controlled signaling pathway and directly switch poly(dC)/RmlB to P-poly(dC)/RmlB or individual RmlB. In response to the switch in the complex physiological state, cells decrease PMF and intracellular ATP level and shutdown the dTDP-l-rhamnose pathway, forming persistence in PAO1 Homologous recombination Supplementary Table 6 listed the primer pairs for amplification of all homologous arms. The upstream and downstream homologous arms were ligated by overlap PCR and inserted into pEX18Gm. The resulting plasmid was transformed into E. coli SM10 ( λ pir ) and then transferred into P. aeruginosa PAO1 by parental mating. Single cross-over recombinant were selected from LB agar plus 50 μg ml −1 gentamicin and 60 μg ml −1 ampicillin and further cultured on fresh LB agar containing 20% sucrose for screening the phenotypes of sucrose R recombinants (double cross-over). In rmlA , rmlB , rmlC , and rmlD knockout experiments, 1 mg ml −1 rhamnose was extra added to both recombinant screening media to support mutant growth. Measurement of PMF PMF was estimated using DiBAC 4 (3) [43] , [44] , [45] . Samples were centrifuged at 12,000 × g for 3 min at room temperature for removal of phenazine pyocyanin. The collected cells (without washing) were diluted to 10 5 CFU ml −1 in PBS with 10 μM DiBAC 4 (3) and then incubated at room temperature for 10 min. The cells were analyzed by a BD Accuri C6 Flow Cytometer equipped with a 488 nm (green) laser and 530 nm filter. ATP assay Cells were centrifuged at 12,000 × g for 3 min at room temperature and washed in 50 mM Tris-acetate, pH 7.75. ATP was extracted by 1% TCA in Tris-acetate buffer at 4 °C for 10 min. 1 ml Tris-acetate buffer was added to obtain a pH of 7.75 before mixing with rL/L reagent (ENLITEN ATP assay, Promega) at room temperature. The amount of ATP extracted was calculated from values obtained with a Bio-orbit 1253 luminometer (Bio-orbit Oy) using dilutions of known amounts of ATP for a standard curve according to the manufacturer’s protocol. Assay of the activity of dTDP- d -glucose 4,6-dehydratase The activity of dTDP- d -glucose 4,6-dehydratase was determined by incubation of His-tagged RmlB, poly(dC 12 )/His-tagged RmlB or P-poly(dC 12 )/His-tagged RmlB with 0.1 mM dTDP- d -glucose in 50 mM Hepes (pH 7.5) plus 10% glycerol, 0.01 mM NADH, and 0.1 mM MgCl 2 at 37 °C for 30 min. The free and ssDNA bound His-tagged RmlB were 12 μg μl −1 , respectively. Both complexes were prepared as described in EMSA section. All reaction mixtures were then analyzed by an Agilent 1260 high-performance liquid chromatography (HPLC) equipped with a Nova-Par C 18 column (3.9 × 150 mm). KH 2 PO 4 (500 mM) was used as mobile phase with a flow rate of 0.8 ml min −1 at 25 °C. The substrate dTDP- d -glucose was monitored at 254 nm. Intracellular free l -rhamnose assay Cells were harvested, resuspended in an equal volume of 10 mM PBS (pH 7.5), and disrupted by sonication. The concentration of free l -rhamnose was then detected by using the l -Rhamnose Assay Kit (Megazyme). Quantification and statistical analysis Statistical parameters including the exact value of n , SD and statistical significance are reported in the figures and the figure legends. Statistical significance is determined by the value of P < 0.05 by two-tailed Student’s t -test, where appropriate.